Significant contributions of combustion-related sources to ammonia emissions Atmospheric ammonia (NH 3 ) and ammonium (NH 4 + ) can substantially influence air quality, ecosystems, and climate. NH 3 volatilization from fertilizers and wastes (v-NH 3 ) has long been assumed to be the primary NH 3 source, but the contribution of combustion-related NH 3 (c-NH 3 , mainly fossil fuels and biomass burning) remains unconstrained. Here, we collated nitrogen isotopes of atmospheric NH 3 and NH 4 + and established a robust method to differentiate v-NH 3 and c-NH 3 . We found that the relative contribution of the c-NH 3 in the total NH 3 emissions reached up to 40 ± 21% (6.6 ± 3.4 Tg N yr −1 ), 49 ± 16% (2.8 ± 0.9 Tg N yr −1 ), and 44 ± 19% (2.8 ± 1.3 Tg N yr −1 ) in East Asia, North America, and Europe, respectively, though its fractions and amounts in these regions generally decreased over the past decades. Given its importance, c-NH 3 emission should be considered in making emission inventories, dispersion modeling, mitigation strategies, budgeting deposition fluxes, and evaluating the ecological effects of atmospheric NH 3 loading. Ammonia (NH 3 ) is a highly water-soluble and reactive gas in the atmosphere [1] . The uptake of NH 3 within clouds and rain and onto atmospheric aerosols causes the formation of ammonium (NH 4 + ) within atmospheric particulates and precipitation (denoted as p-NH 4 + and w-NH 4 + , respectively) [1] , [2] , [3] . Over the last century, urbanization and industrial and agricultural intensification have greatly increased NH 3 production and have led to a continuous increase in the NH 3 emission amounts and deposition fluxes [4] , [5] , [6] , [7] , [8] . Globally, the NH 3 emission has increased from 20.6 Tg N yr −1 in 1860 to 58.2 Tg N yr −1 in 1993 and may double to 118.0 Tg N yr −1 by 2050 [4] . 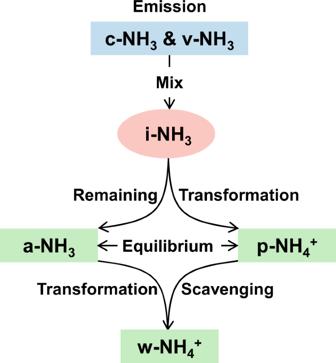Fig. 1: Conceptual framework of atmospheric NH3and NH4+. It shows the relationships among NH3emissions from combustion-related sources (c-NH3) and volatilization sources (v-NH3), the initial mixture of c-NH3and v-NH3(i-NH3), ambient NH3(a-NH3), particulate NH4+(p-NH4+), and precipitation NH4+(w-NH4+). The a-NH3potentially includes the NH3that has not been converted to p-NH4+in earlier stages and the fresh NH3emissions in relatively later periods. Since the 1950s, East Asia, North America, and Europe have been three regions of high NH 3 emissions [9] , [10] , with total emission amounts of 10.7 ± 0.4, 3.7 ± 0.2, and 3.5 ± 0.3 Tg N yr −1 during 2000–2015, respectively, according to emission inventory data (Supplementary Table 1 ). As a result, atmospheric NH 3 concentrations (averaging 2.9 ± 2.4, 1.4 ± 1.8, 1.2 ± 1.3 μg m −3 , respectively [11] ) and NH x deposition (the sum of NH 3 , p-NH 4 + , and w-NH 4 + ) (averaging 12.0, 4.7, and 6.9 Tg N yr −1 , respectively [12] , [13] ) in the above three regions also remain high. In human-disturbed areas, excessive NH 3 has promoted secondary aerosol production and air pollution [2] , [3] , [4] . Elevated NH x concentrations and deposition have caused negative impacts on ecosystem structure and function (e.g., biodiversity declines, soil acidification, water eutrophication [2] , [3] , [14] ) and huge economic loss [15] , [16] , [17] . There are two major groups of atmospheric NH 3 emission sources. One is NH 3 volatilization from NH 4 + -containing substrates (mainly fertilized and natural soils, animal wastes, and natural and N-polluted water) (denoted as v-NH 3 ) [2] , [9] , [18] , [19] . The dissolved NH 3 volatilizes from liquid-phase substrates containing NH 4 + at favorable pH, temperature, and pressure conditions [20] . The other is NH 3 emission from combustion-related sources (mainly coal combustion, vehicle exhausts, and biomass burning) (denoted as c-NH 3 ) [21] , [22] , [23] , [24] . NH 3 would be released from industrial coal combustion, heavy-duty and light-duty diesel vehicles equipped with selective catalytic or non-catalytic reduction systems because of excessive urea/NH 3 used for the catalytic degradation of nitrogen oxides (NO x ) [25] , [26] . It is also produced via steam reforming from hydrocarbons [27] and or catalytic reaction of nitric oxide with molecular hydrogen [28] in light and medium-dust gasoline vehicles equipped with three-way catalytic converters, relating to the catalyst temperatures and air-to-fuel ratios [29] . The biomass N, typically as amides (R-(C = O)-NH-R’) and amines (R-NH 2 ), can produce NH 3 under poor mixing conditions during biomass burning [30] . So far, there have been direct observations on emission factors of various v-NH 3 sources to budget the v-NH 3 emission amount (Supplementary Table 1 ; Supplementary Fig. 1a ). According to statistical emission inventories, the v-NH 3 is the dominant source of regional NH 3 emissions, accounting for 94 ± 1%, 90 ± 1%, and 95 ± 1% of the total emission in East Asia during 2001–2015, North America during 1970–2019, and Europe during 1970–2018, respectively (Supplementary Fig. 1b ). In contrast, it has long been difficult to estimate the c-NH 3 emission because of limited data on emission factors of c-NH 3 sources and uncertainties associated with the amount of combusted materials, especially biomasses [22] , [23] . 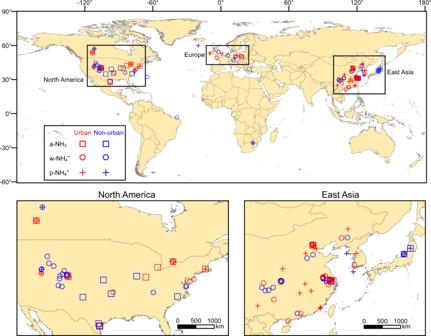Fig. 2: Global and regional maps with the observation sites forδ15N of ambient NH3(a-NH3), particulate NH4+(p-NH4+), and precipitation NH4+(w-NH4+) in East Asia, North America, and Europe. Maps were created by using ArcGIS version 10.5 (Esri Inc., USA). The base map was download fromhttps://hub.arcgis.com/datasets/esri::world-countries-generalized. However, evidence from laboratory simulations, in-situ observations, satellite observations, and emission inventories points to an underestimation of c-NH 3 emissions relative to previous assessments (summarized in Supplementary Table 2 ). First, laboratory simulations found that biomass burning and light-duty diesel vehicles equipped with selective catalytic reduction are important NH 3 sources and have been overlooked (Supplementary Table 2 ). Second, ground observations found that ambient NH 3 concentrations at sites impacted by biomass burning, traffic pollution, industrial pollution, or urban pollution were enhanced by a factor of 1.4–20 compared to unpolluted sites (Supplementary Table 2 ). Third, satellite observations revealed that the NH 3 from biomass burning controlled seasonal variations of surface NH 3 concentrations in the southern and high-emission regions of China, the USA, and Europe in the northern hemisphere (Supplementary Table 2 ). Spatially, satellite observations also identified 13 hotspots of urban NH 3 pollution and 266 hotspots of industrial NH 3 pollution from coal combustion and coal-related industries (Supplementary Table 2 ). Fourth, according to emission inventories, the total c-NH 3 emissions from transportation (1.3 Tg N yr −1 ) [23] , biomass burning (8.2 Tg N yr −1 ) [31] , and other combustion sources (6.3 Tg N yr −1 ) [10] has reached up to 15.9 Tg N yr −1 , which accounts for 30% of the global NH 3 emission (54.3 Tg N yr −1 ). Additionally, isotopic evidence demonstrated that c-NH 3 had reached 29–62% in NH 3 of the ambient atmosphere [32] , [33] , [34] and 45–90% of the NH 4 + deposition in cities of China and the USA [35] , [36] . All the above evidence suggests that the relative importance and amount of regional c-NH 3 emissions are still open questions and should be re-evaluated. Here we collated observation data of natural N isotopes (expressed as δ 15 N, δ 15 N = ( 15 N / 14 N) sample /( 15 N / 14 N) standard −1, where atmospheric N 2 is used as the standard) of primary v-NH 3 and c-NH 3 emission sources (Supplementary Fig. 2 ), NH 3 gas in the ambient atmosphere (a-NH 3 ), NH 4 + in atmospheric particulates (p-NH 4 + ) and precipitation (w-NH 4 + ) in East Asia, North America, and Europe (Fig. 1 – 3 ; Supplementary Figs. 3 & 4 ). In combination with the collected data of a-NH 3 and p-NH 4 + concentrations observed in the above regions, we evaluated δ 15 N differences of the initial NH 3 mixture of v-NH 3 and c-NH 3 (i-NH 3 ) to a-NH 3 , p-NH 4 + , or w-NH 4 + , respectively (Supplementary Figs. 5 – 9 ; detailed in Methods). Then, based on the source δ 15 N, δ 15 N difference, δ 15 N observation of a-NH 3 , p-NH 4 + , and w-NH 4 + , and the Stable Isotope Analysis in R model (i.e., the SIAR model; detailed in Methods), we established a set of isotopic methods to calculate relative contributions between v-NH 3 and c-NH 3 in above study regions (Fig. 4 & 5 ; Supplementary Figs. 10 – 12 ). Finally, using regional mean fraction values and emission amounts of v-NH 3 , we recalculated the amounts of c-NH 3 and total NH 3 emissions in each region (Fig. 5 ; Supplementary Figs. 13 & 14 ). Fig. 1: Conceptual framework of atmospheric NH 3 and NH 4 + . It shows the relationships among NH 3 emissions from combustion-related sources (c-NH 3 ) and volatilization sources (v-NH 3 ), the initial mixture of c-NH 3 and v-NH 3 (i-NH 3 ), ambient NH 3 (a-NH 3 ), particulate NH 4 + (p-NH 4 + ), and precipitation NH 4 + (w-NH 4 + ). The a-NH 3 potentially includes the NH 3 that has not been converted to p-NH 4 + in earlier stages and the fresh NH 3 emissions in relatively later periods. Full size image Fig. 2: Global and regional maps with the observation sites for δ 15 N of ambient NH 3 (a-NH 3 ), particulate NH 4 + (p-NH 4 + ), and precipitation NH 4 + (w-NH 4 + ) in East Asia, North America, and Europe. Maps were created by using ArcGIS version 10.5 (Esri Inc., USA). The base map was download from https://hub.arcgis.com/datasets/esri::world-countries-generalized . Full size image Fig. 3: δ 15 N of ambient NH 3 (a-NH 3 ), particulate NH 4 + (p-NH 4 + ), and precipitation NH 4 + (w-NH 4 + ) (a) and the initial NH 3 mixture from different sources ( δ 15 N i-NH3 ) (b) in East Asia, North America, and Europe. Each data point represents the site-based mean δ 15 N. Each box encompasses the 25 th −75 th percentiles, whiskers and red lines in boxes are the SD and mean values, respectively. The number below each box is that of observation sites. Note that the site with simultaneous a-NH 3 , w-NH 4 + , or p-NH 4 + observation is counted as one site in sub-figure b. In sub-figure a, different letters ( a, b, and c ) above the boxes indicate the significant differences ( p < 0.05) among species in the same region; in sub-figure b, different letters ( a and b ) above the boxes indicate the significant differences among the three regions. The δ 15 N a-NH3 based on the passive samplers have been calibrated by adding 15‰ [41] . The δ 15 N i-NH3 was calculated according to Eqs. ( 11 – 13 ) (detailed in Methods). Full size image Fig. 4: Temporal variations of δ 15 N of the initial NH 3 mixture from different sources ( δ 15 N i-NH3 ) in East Asia, North America, and Europe. The mean ± SD of replicate measurements at each site in each year is shown. We counted the same site with different years as different observations, given that δ 15 N observations at a few sites have been conducted in different sampling years. Full size image Fig. 5: Relative contributions of volatilization NH 3 (v-NH 3 ) and combustion-related NH 3 (c-NH 3 ) sources (a) and their emission amounts (b). The ‘Total’ is the sum of v-NH 3 and c-NH 3 . Mean±SD is shown. Full size image δ 15 N signatures of v-NH 3 and c-NH 3 δ 15 N for v-NH 3 ( δ 15 N v-NH3 ) average −18.9 ± 4.2‰, significantly lower than c-NH 3 ( δ 15 N c-NH3 , averaging 8.0 ± 4.4‰) (Supplementary Fig. 2b , detailed in Methods). The volatilization of NH 3 includes three main steps, i.e., the equilibrium of NH 4 + ↔ NH 3 , the diffusion of NH 3 to and away from volatilization sites [37] . The overall isotope effects range from −60‰ to −30‰ (depending on temperature, pH, and cation-exchange capacities of substrates [20] , [38] , [39] , [40] , causing the low δ 15 N v-NH3 . Differently, δ 15 N c-NH3 would assemble or be slightly higher than δ 15 N of burning materials that are relatively 15 N-enriched [41] . Distinct δ 15 N v-NH3 and δ 15 N c-NH3 provide a unique tool to differentiate the relative contributions between v-NH 3 and c-NH 3 in the SIAR isotope mass-balance model. δ 15 N differences between a-NH 3 , p-NH 4 + , or w-NH 4 + and i-NH 3 The δ 15 N of the initial NH 3 mixture of v-NH 3 and c-NH 3 emissions ( δ 15 N i-NH3 ) integrate their δ 15 N signatures and fractional contributions ( F v-NH3 and F c-NH3 , respectively) (Fig. 1 , Eq. ( 1 )). δ^15N_i-NH3=δ^15N_v-NH3×F_v-NH3+δ^15N_c-NH3×F_c-NH3
 (1) where F v-NH3 + F c-NH3 = 1. However, because NH 3 is very reactive and readily transformed into NH 4 + , it is difficult in reality, if not impossible, to directly measure δ 15 N i-NH3 [42] , [43] . Practically, site-based δ 15 N values of a-NH 3 , p-NH 4 + , and w-NH 4 + have been widely measured (Fig. 2 ). However, their δ 15 N, namely δ 15 N a-NH3 , δ 15 N p-NH4+ , and δ 15 N w-NH4+ , cannot be directly used as δ 15 N i-NH3 to calculate F v-NH3 and F c-NH3 (Eq. ( 1 )). First, the i-NH 3 mixture of v-NH 3 and c-NH 3 emissions will be partially converted to p-NH 4 + and w-NH 4 + (Fig. 1 ). 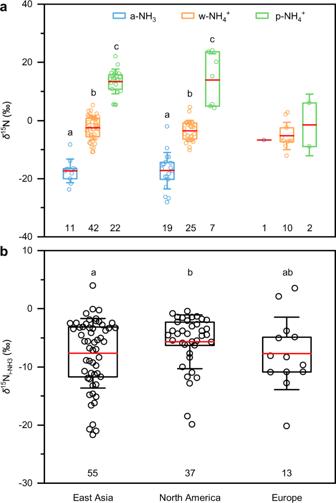Fig. 3:δ15N of ambient NH3(a-NH3), particulate NH4+(p-NH4+), and precipitation NH4+(w-NH4+) (a) and the initial NH3mixture from different sources (δ15Ni-NH3) (b) in East Asia, North America, and Europe. Each data point represents the site-based meanδ15N. Each box encompasses the 25th−75thpercentiles, whiskers and red lines in boxes are the SD and mean values, respectively. The number below each box is that of observation sites. Note that the site with simultaneous a-NH3, w-NH4+, or p-NH4+observation is counted as one site in sub-figure b. In sub-figure a, different letters (a, b,andc) above the boxes indicate the significant differences (p< 0.05) among species in the same region; in sub-figure b, different letters (aandb) above the boxes indicate the significant differences among the three regions. Theδ15Na-NH3based on the passive samplers have been calibrated by adding 15‰41. Theδ15Ni-NH3was calculated according to Eqs. (11–13) (detailed in Methods). The conversion of NH 3 to p-NH 4 + has significant isotope effects as a result of either kinetic isotope fractionations ( ε k ) during the unidirectional reaction of NH 3 → p-NH 4 + or equilibrium isotope fractionations ( ε eq ) during reversible reactions of NH 3 ↔ p-NH 4 + (Supplementary Table 3 ). Accordingly, δ 15 N a-NH3 and δ 15 N p-NH4+ differ from δ 15 N i-NH3 and thus cannot be directly used in Eq. ( 1 ) [34] , [35] . Second, precipitation scavenges both a-NH 3 and p-NH 4 + via the rainout and washout processes (Fig. 1 ), but the preferential wet scavenge between a-NH 3 and p-NH 4 + can potentially cause differences between δ 15 N w-NH4+ and δ 15 N i-NH3 [44] . Consequently, δ 15 N w-NH4+ cannot be directly used to calculate F v-NH3 and F c-NH3 in Eq. ( 1 ) either. 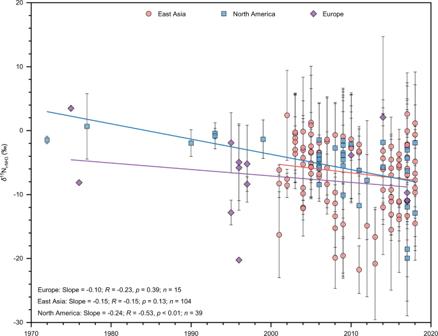Fig. 4: Temporal variations ofδ15N of the initial NH3mixture from different sources (δ15Ni-NH3) in East Asia, North America, and Europe. The mean ± SD of replicate measurements at each site in each year is shown. We counted the same site with different years as different observations, given thatδ15N observations at a few sites have been conducted in different sampling years. According to both simultaneous observations at the same sites (Supplementary Table 4 ) and non-synchronous observations in the same regions (Fig. 3a ), δ 15 N in NH 4 + (particularly p-NH 4 + ) are generally higher than δ 15 N a-NH3 , which is generally negative (Fig. 3a ). The main reason is that large equilibrium isotope fractionations occur during the transformation of NH 3 to NH 4 + (Supplementary Table 3 ), leading to substantial differences (denoted as 15 ∆ ) of δ 15 N a-NH3 , δ 15 N p-NH4+ , or δ 15 N w-NH4+ to the corresponding δ 15 N i-NH3 ( 15 ∆ a-NH3 , 15 ∆ p-NH4+ , and 15 ∆ w-NH4+ , respectively). In this work, we developed a new set of methods to constrain 15 ∆ a-NH3 , 15 ∆ p-NH4+ , and 15 ∆ w-NH4+ , and then reconstruct δ 15 N i-NH3 (detailed in Methods). 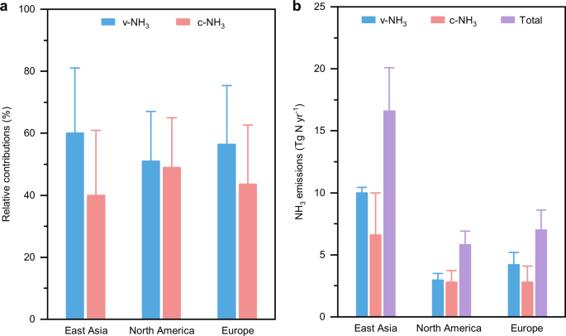Fig. 5: Relative contributions of volatilization NH3(v-NH3) and combustion-related NH3(c-NH3) sources (a) and their emission amounts (b). The ‘Total’ is the sum of v-NH3and c-NH3. Mean±SD is shown. Generally, based on simultaneous observation data of seasonal mean C a-NH3 , C p-NH4+ , δ 15 N a-NH3 , δ 15 N p-NH4+ , and δ 15 N w-NH4+ at six sites (Supplementary Table 5 ), we estimated corresponding δ 15 N i-NH3 , 15 ∆ a-NH3 , 15 ∆ p-NH4+ , and 15 ∆ w-NH4+ (Eqs. ( 7 – 10 ); detailed in Methods). Then, we established the relationships between 15 ∆ a-NH3 , 15 ∆ p-NH4+ , or 15 ∆ w-NH4+ and atmospheric NH 3 conversion ratios (expressed as f p-NH4+ , i.e., C p-NH4+ /( C a-NH3 + C p-NH4+ )) (Supplementary Fig. 5 ). These relationships show that 15 ∆ a-NH3 , 15 ∆ p-NH4+ , and 15 ∆ w-NH4+ decrease with an increase of f p-NH4+ (Supplementary Fig. 5 ). 15 ∆ a-NH3 and 15 ∆ p-NH4+ vary linearly with the reaction degree of an open system (i.e., f p-NH4+ ) (Supplementary Fig. 5a ) consistent with the prediction of isotopic theory [45] . The 15 ∆ w-NH4+ includes 15 ∆ a-NH3 and 15 ∆ p-NH4+ because precipitation scavenges a-NH 3 and p-NH 4 + via the rainout and washout processes (Supplementary Fig. 5b ). Meanwhile, we examined the impact of historical NO x and sulfur dioxide (SO 2 ) reductions on mean annual f p-NH4+ (Supplementary Fig. 6a–f ). The f p-NH4+ generally decreased from 1990 to 2017 in Europe and 2004 to 2018 in North America, but did not vary clearly from 2000 to 2018 in East Asia (Supplementary Fig. 7 ). Then, based on the relationships between 15 ∆ a-NH3 , 15 ∆ p-NH4+ , or 15 ∆ w-NH4+ and f p-NH4+ (Supplementary Fig. 5 ) and mean annual f p-NH4+ values (Supplementary Fig. 7 ), we calculated mean annual 15 ∆ a-NH3 , 15 ∆ p-NH4+ , and 15 ∆ w-NH4+ in each region (Supplementary Fig. 8 ), which were further used to calculate the corresponding δ 15 N i-NH3 (Fig. 3b ) of site-based δ 15 N a-NH3 , δ 15 N p-NH4+ , or δ 15 N w-NH4+ (Fig. 3a ) (detailed in Methods). Spatial and temporal patterns of δ 15 N i-NH3 variations Spatially, δ 15 N i-NH3 is higher in North America (−5.7 ± 4.6‰) than in Europe (−7.7 ± 6.3‰) and East Asia (−8.0 ± 6.0‰) (Fig. 3b ). Because the δ 15 N c-NH3 is distinctly higher than the δ 15 N v-NH3 (Supplementary Fig. 2 ), the emission strength of c-NH 3 relative to v-NH 3 in North America is higher than that in East Asia and Europe. On the one hand, the emission inventories also show that the proportion of v-NH 3 in North America is lower than that in East Asia and Europe (Supplementary Fig. 1b ). On the other hand, because energy consumption is the primary source of c-NH 3 and fertilizer consumption and animal manure are the source of v-NH 3 (Supplementary Fig. 15a, b ), the energy consumption ratio to fertilizer consumption and animal manure is higher in North America than in East Asia and Europe (Supplementary Fig. 15c ). δ 15 N i-NH3 decreased significantly between 1972 and 2018 in North America ( p < 0.01) and decreased slightly from 2001 to 2018 in East Asia ( p = 0.13) and 1974–2017 in Europe ( p = 0.39) (Fig. 4 ). These results suggest that the emission strength of v-NH 3 relative to c-NH 3 generally increased during the past decades in our three study regions, especially in North America. This finding coincided with increasing fertilizer consumption and animal manure in East Asia and North America over the past decades (Supplementary Fig. 16 ). Relative contributions and amounts of v-NH 3 and c-NH 3 emissions We considered 15 ∆ a-NH3 , 15 ∆ p-NH4+ , and 15 ∆ w-NH4+ (detailed in Methods) in Eq. ( 1 ) to establish a set of new isotope mass-balance equations to calculate F v-NH3 and F c-NH3 by using δ 15 N a-NH3 , δ 15 N p-NH4+ , or δ 15 N w-NH4+ in each region (Eqs. ( 2 – 4 ), respectively). δ^15N_a-NH3=δ^15N_v-NH3×F_v-NH3+δ^15N_c-NH3×F_c-NH3+^15 _a-NH3
 (2) 
    δ^15N_p-NH4+=δ^15N_v-NH3×F_v-NH3+δ^15N_c-NH3×F_c-NH3+^15 _p-NH4+
 (3) 
    δ^15N_w-NH4+=δ^15N_v-NH3×F_v-NH3+δ^15N_c-NH3×F_c-NH3+^15 _w-NH4+
 (4) F v-NH3 and F c-NH3 values were calculated by the SIAR model (detailed in Methods). F c-NH3 averages 40 ± 21% in East Asia, 49 ± 16% in North America, and 44 ± 19% in Europe (Fig. 5a ), which confirms higher emission strength of c-NH 3 relative to v-NH 3 in North America than in East Asia and Europe. These estimations based on isotope methods are generally higher than the fractions of c-NH 3 emissions in corresponding regions (5–10%; Supplementary Fig. 1b ) or the globe based on emission inventories (30% [10] , [23] , [31] ). One possible explanation is that the study regions are hotspots of globally high c-NH 3 emissions [24] . Supportively, the total consumption of fossil fuels in these regions accounts for more than 60% of the global energy consumption (Supplementary Fig. 15a ), though their areas account for only 24% of the worldwide land area [46] . Further, the spatial pattern of F c-NH3 (North America > Europe > East Asia; Fig. 5a ) assembles that of the energy consumption ratio to fertilizer consumption and animal manure (Supplementary Fig. 15c ). Based on F v-NH3 in our study and explicit amounts of v-NH 3 ( A v-NH3 ) in emission inventories (Fig. 5 ), we further estimated the amounts of c-NH 3 ( A c-NH3 ) and total NH 3 emissions (detailed in Methods), which average 6.6 ± 3.4 Tg N yr −1 and 16.6 ± 3.5 Tg N yr −1 in East Asia, 2.8 ± 0.9 Tg N yr −1 and 5.8 ± 1.1 Tg N yr −1 in North America, and 2.8 ± 1.3 Tg N yr −1 and 7.0 ± 1.6 Tg N yr −1 in Europe, respectively (Fig. 5b ). The highest energy consumption in East Asia supports its highest A c-NH3 among the three study regions (Fig. 5b & Supplementary Fig. 15a ). Our new estimates of total NH 3 emission in Europe are very close to its total NH x deposition (Supplementary Fig. 13 ). In China and the United States, the NH x deposition fluxes could be explained by our updated total NH 3 emissions (Supplementary Fig. 13 ). Lower deposition than the emission was observed in China and the United States because part of the NH 3 emissions was diffused or deposited out of these polluted areas [24] , [47] . Before this work, total NH 3 emissions based on statistical inventories in China, the United States, and Europe were all distinctly lower than the corresponding NH x deposition (Supplementary Fig. 13 ). Accordingly, our results provided new estimates on c-NH 3 and total NH 3 emissions. However, because the v-NH 3 underestimation may still exist [48] , the contribution of the c-NH 3 underestimation to the underestimation of total NH 3 emissions and the mismatches between regional NH 3 emissions and NH x deposition (Supplementary Fig. 13 ) remains uncertain. Temporally, F c-NH3 has decreased significantly ( p < 0.01) over the past decades in North America (Supplementary Fig. 12a ), leading to increasing ratios of F v-NH3 to F c-NH3 ( p < 0.01) and also A v-NH3 to A c-NH3 ( p < 0.05) generally from lower than 1.0 to higher than 1.0 (Supplementary Figs. 12b & 14b ). F c-NH3 in East Asia and Europe has decreased slightly ( p = 0.12 and p = 0.26, respectively) (Supplementary Fig. 12a ), leading to slightly increasing ratios of F v-NH3 to F c-NH3 ( p = 0.12 and p = 0.51, respectively) and also A v-NH3 to A c-NH3 over the past decades ( p = 0.25 and p = 0.61, respectively) (Supplementary Figs. 12b & 14b ). In East Asia and North America, the temporally increasing v-NH 3 emissions relative to c-NH 3 are supported by the increasing fertilizer consumption and animal manure production (Supplementary Fig. 16 ). Emission inventories also showed the rapid increase of the relative contribution of v-NH 3 in North America (Supplementary Fig. 1b ). These temporal variations in North America revealed that the more dominant NH 3 emission has shifted from c-NH 3 to v-NH 3 sources over the past decades. Rapidly increasing v-NH 3 emissions may be one of the reasons for the shift from nitrate-dominated to NH 4 + -dominated N deposition in the United States [7] . In this study, the non-urban F c-NH3 does not change with the corresponding distance between the sampling site and the nearest urban area (Supplementary Fig. 11 ). Meanwhile, there are no significant differences in F c-NH3 between urban (73 sites) and non-urban (65 sites) or between agricultural (32 sites) and non-agricultural sites (33 sites) (Supplementary Fig. 11 ). Similar numbers of replicate sites between the above surface environments reduce the risks of over- or under-estimating c-NH 3 or v-NH 3 contributions. Accordingly, the F c-NH3 at urban or non-urban sites is not substantially influenced by local NH 3 emissions but reflects the source diversity and transporting/mixing complexity of regional NH 3 emissions. There has been much evidence from ground monitoring, satellite observations, and emission inventories to show the co-occurrence of c-NH 3 and v-NH 3 emissions and extensive NH 3 or NH 4 + transportation and mixing among landscapes. Firstly, v-NH 3 sources (mainly from solid wastes and sewages) have comparable emission strengths with c-NH 3 sources (mainly from fossil fuel combustion) in urban areas. Human excreta contributed 11.4% to the total NH 3 emissions in Shanghai urban of eastern China [49] . The v-NH 3 from urban green space contributed up to 60% to ambient NH 3 in Qingdao in northern China [50] . The urban NH 3 concentrations influenced by the v-NH 3 from urban waste containers, sewage systems, humans, and open markets were 2.5 times higher than that of traffic-influenced urban areas in Spain [51] . Ambient NH 3 concentrations in the Beijing urban peaked when fertilizer was intensively applied on the North China Plain [52] . Secondly, the c-NH 3 emission (mainly wildfire, fossil fuel and crop residue combustion) is undoubtedly as significant as the v-NH 3 (mainly fertilizer application and live stocks) in non-urban areas. For example, the c-NH 3 from biomass burning control seasonal variations of surface NH 3 concentrations in major disturbed regions of the Northern Hemisphere, which is even stronger in the Southern Hemisphere with frequent wildfires (Supplementary Table 2 ). Based on a data synthesis (Supplementary Table 2 ), ambient NH 3 concentrations during wildfire smoke-impacted periods could be enhanced by a factor of 2–20 compared to periods with no wildfires. Besides, our results, as well as previous studies, show that v-NH 3 contributed 58% (31–87%) for sites in Beijing urban [34] , [35] , [53] , while the c-NH 3 accounted for 33% (25–69%) in the total NH 4 + deposition of the cropland 370 km far from the Beijing urban [11] . Collectively, site-based δ 15 N a-NH3 and δ 15 N NH4+ represent mixing signatures and can be feasibly used to evaluate regional c-NH 3 and v-NH 3 emissions. Implications and uncertainties This study demonstrates that c-NH 3 emissions have been considerably underestimated in regions with significant anthropogenic sources. In the process, the new estimates of c-NH 3 emissions have brought measured NH x deposition data into closer agreement with emissions. Our conclusion about the underestimation of c-NH 3 emission has important implications for control measures since the current efforts have been focused almost exclusively on agricultural sources. Although the marginal abatement cost of NH 3 emissions is only 10% of the global NO x emission, with 162 billion US dollars net benefit, the reduction can effectively improve air pollution and its negative impact [54] , [55] . For example, measures to reduce c-NH 3 emissions should be considered in the methods for mitigating v-NH 3 emissions by improved farm management practices with N use reductions, deep machine placement of fertilizer, enhanced-efficiency fertilizer use, and enhanced manure management in the agriculture sector [56] , [57] . The revelation of high c-NH 3 emissions also implies that the potential, costs, and impacts of NH 3 emissions reduction need to be re-assessed. Steps to reduce c-NH 3 emissions may alleviate the pressure of reducing agricultural NH 3 emissions and achieve ‘win-win’ outcomes for agricultural production and food supply, human and environmental health [2] , [56] . The uncertainty of this study lies in the technical difficulty in measuring δ 15 N for all NH 3 emission sources in each region. It is even more challenging to conduct simultaneous observations on C a-NH3 , C p-NH4+ , δ 15 N a-NH3 , δ 15 N p-NH4+ , and δ 15 N w-NH4+ among landscapes. As a result, a limited number of data is available in terms of observation sites and their spatial distribution in the three regions, and the corresponding data comparison among the three regions is preliminary in the current stage. Moreover, δ 15 N observations focus largely on the middle- and low-latitudes and low altitudes of the Northern Hemisphere but rare on the high mountains and high latitudes of the Northern Hemisphere and the Southern Hemisphere. More observations on the concentration and δ 15 N parameters of NH 3 and NH 4 + in both source emissions and deposition are necessary to improve the isotope source apportionment, especially in remote areas. Finally, despite the updated regional c-NH 3 and total NH 3 emissions, future in-depth cooperation among different observational and modeling methods should be encouraged. δ 15 N of major NH 3 emission sources We collected the δ 15 N data of major NH 3 emission sources (Supplementary Fig. 2a ) from 17 relevant publications (by December 2020). For c-NH 3 , the proportional contributions of global NH 3 emissions from vehicle exhausts (ve-NH 3 ), coal combustion (cc-NH 3 ), and biomass burning (bb-NH 3 ) (1.3, 6.3, and 8.2 Tg N yr −1 , respectively [10] , [23] , [31] ) in total c-NH 3 emissions (15.9 Tg N yr −1 ) are 8%, 40%, and 52%, respectively (Eq. ( 5 )). Accordingly, we calculated the δ 15 N c-NH3 by a mass-balance method (Eq. ( 5 )). δ^15N_c-NH3=δ^15N_ve-NH3× 8 %+δ^15N_cc-NH3× 40%+δ^15N_bb-NH3× 52%
 (5) For v-NH 3 , global NH 3 emissions from fertilizer application (fa-NH 3 ) and waste materials (wm-NH 3 ) account for 56% and 44% of the total v-NH 3 emission, respectively [10] . Similarly, we calculated the δ 15 N v-NH3 by Eq. ( 6 ). δ^15N_v-NH3=δ^15N_fa-NH3× 56%+δ^15N_wm-NH3× 44%
 (6) The standard deviation (SD) of δ 15 N c-NH3 and δ 15 N v-NH3 is propagated errors estimated using the Monte Carlo method (MCM). Briefly, we ran 10000 trials for the MCM in the software of Microsoft Excel-Add-In and calibrated the SD to match the corresponding true values. Atmospheric δ 15 N a-NH3 , δ 15 N p-NH4+ , and δ 15 N w-NH4+ observations Keywords used for the search are ‘nitrogen isotope’, ‘ammonia/NH 3 ’, ‘ammonium/NH 4 + ’, ‘rainfall’, ‘rain’, ‘rain water’, ‘precipitation’, ‘aerosol’, and ‘particulate’. The databases include the Web of Science ( http://isiknowledge.com ), Google Scholar ( http://scholar.google.com.hk ), and Baidu Scholar ( http://xueshu.baidu.com ). By December 2020, there are 18 publications on δ 15 N a-NH3 (listed in Supplementary Text 1 ), 43 publications on δ 15 N w-NH4+ (listed in Supplementary Text 2 ), and 28 publications on δ 15 N p-NH4+ (listed in Supplementary Text 3 ). Data in the figures of these publications were extracted using the software of Web Plot Digitizer (Version 4.2, San Francisco, California, USA). Spatial distributions of the sites with δ 15 N a-NH3 , δ 15 N p-NH4+ , and δ 15 N w-NH4+ observations are shown in Fig. 2 . When counting the same site with observations in different years as one site only, there are 387 measurements of δ 15 N a-NH3 at 32 sites (including 12 sites in East Asia, 19 sites in North America, and one site in Europe), 857 measurements of δ 15 N p-NH4+ at 33 sites (including 22 sites in East Asia, seven sites in North America, two sites in Europe, one site in Africa, and one site in Atlantic), and 1540 measurements of δ 15 N w-NH4+ at 80 sites (including 42 sites in East Asia, 25 sites in North America, ten sites in Europe, one site in South America, one site in Africa, and one site in Atlantic) (Fig. 2 & Supplementary Fig. 3 ). The surface land types of observation sites were identified according to descriptions in original publications. There are 73 urban sites (mainly constructed lands) and 65 non-urban sites (mainly including 32 agricultural sites and 33 non-agricultural sites) with δ 15 N a-NH3 , δ 15 N p-NH4+ , or δ 15 N w-NH4+ observations in the study areas of East Asia, North America, and Europe (Supplementary Fig. 4a, b ). We only analyzed the data in the major areas of East Asia during 2001–2018, North America during 1972–2018, and Europe during 1974–2017 due to the sparsity of available data out of these areas (Fig. 2 & 4 ). It should be noted that analytical methods of 15 N a-NH3 , δ 15 N p-NH4+ , and δ 15 N w-NH4+ differ among studies, including converting to 1) N 2 as an end product using the Elemental Analyzer combustion method or 2) N 2 O as an end product using the bromate oxidation and azide or hydroxylamine reduction, or using the persulfate oxidation and denitrifier method [58] , but such difference would not change the spatiotemporal patterns of δ 15 N i-NH3 (Fig. 3 & 4 ) because the analytical accuracy is generally better than ±0.7‰. In addition, 9%, 16%, and 75% of the δ 15 N observations were conducted across cooler seasons, warmer seasons, and the whole year, respectively. The seasonal differences in NH 3 emissions would not substantially influence the spatiotemporal patterns of δ 15 N i-NH3 (Fig. 3 & 4 ). Moreover, all observation sites in this study are more than 1 km away from obvious local emission sources, excluding the influence of a single source. Atmospheric C a-NH3 and C p-NH4+ observations ‘Atmospheric ammonia/NH 3 ’, ‘particulate ammonium/NH 4 + ’, and ‘aerosol ammonium/NH 4 + ’ were used as keywords to search publications for the concentration of a-NH 3 and p-NH 4 + ( C a-NH3 and C p-NH4+ , respectively) in the same databases as described above. There are 107 publications published by July 2021 (listed in Supplementary Text 4 ) with simultaneous observations on C a-NH3 and C p-NH4+ . To describe temporal variations of C p-NH4+ /( C a-NH3 + C p-NH4+ ) values (i.e., f p-NH4+ values) in each region (Supplementary Fig. 7 ), we counted the same site with different years as different observations because few sites observed C a-NH3 and C p-NH4+ for many years. We only used data with an observation period exceeding six months to improve the estimation of annual f p-NH4+ values. According to this criterion, there are 262 sites in East Asia during 1993–2018, 459 sites in North America during 1986–2018, and 1018 sites in Europe during 1981–2017 (Supplementary Fig. 7 ). Differences of δ 15 N a-NH3 , δ 15 N p-NH4+ , or δ 15 N w-NH4+ from i-NH 3 Based on simultaneous observations of seasonal C a-NH3 , C p-NH4+ , δ 15 N a-NH3 , δ 15 N p-NH4+ , and δ 15 N w-NH4+ values at the same sites (Supplementary Table 5 ), we calculated the δ 15 N i-NH3 by the following isotope mass-balance equation (Eq. ( 7 )). δ^15N_i-NH3=δ^15N_a-NH3×f_a-NH3+δ^15N_p-NH4+×f_p-NH4+
 (7) where f a-NH3 = C a-NH3 / ( C a-NH3 + C p-NH4+ ) and f p-NH4+ = C p-NH4+ / ( C a-NH3 + C p-NH4+ ). Then, we calculated the differences between δ 15 N i-NH3 and δ 15 N a-NH3 ( 15 ∆ a-NH3 , Eq. ( 8 )), between δ 15 N i-NH3 and δ 15 N p-NH4+ ( 15 ∆ p-NH4+ , Eq. ( 9 )), between δ 15 N i-NH3 and δ 15 N w-NH4+ ( 15 ∆ w-NH4+ , Eq. ( 10 )) for the same sites with simultaneous observations of seasonal C a-NH3 , C p-NH4+ , δ 15 N a-NH3 , δ 15 N p-NH4+ , and δ 15 N w-NH4+ values (Supplementary Table 5 ). ^15 _a-NH3=δ^15N_a-NH3-δ^15N_i-NH3
 (8) 
    ^15 _p-NH4+=δ^15N_p-NH4+-δ^15N_i-NH3
 (9) 
    ^15 _w-NH4+=δ^15N_w-NH4+-δ^15N_i-NH3
 (10) Based on the relationships in Supplementary Fig. 5 and mean annual f p-NH4+ values in Supplementary Fig. 7 , we calculated the mean annual 15 ∆ a-NH3 , 15 ∆ p-NH4+ , and 15 ∆ w-NH4+ in each region (Supplementary Fig. 8 ). Because no clear trends were observed in f p-NH4+ between 2001–2018 in East Asia and before implementing emission reduction measures in Europe (i.e., 1971–1989 in this study) and in North America (i.e., 1971–2004 in this study) [59] , [60] , [61] (Supplementary Fig. 7 ), we calculated isotope effect values by using the mean f p-NH4+ during above-mentioned years in the corresponding region (Supplementary Fig. 8 ). In other words, the same values are assumed for 15 ∆ a-NH3 , 15 ∆ p-NH4+ , or 15 ∆ w-NH4+ during these years in the region (Supplementary Fig. 8 ). To examine the applicability of our method for estimating and calibrating 15 ∆ values, we used the mean annual 15 ∆ values and simultaneous δ 15 N a-NH3 and δ 15 N p-NH4+ observations, δ 15 N a-NH3 and δ 15 N w-NH4+ observations, or δ 15 N p-NH4+ and δ 15 N w-NH4+ observations at the same sites (Supplementary Table 4 ) to calculate their corresponding δ 15 N i-NH3 (denoted as δ 15 N i-NH3(a-NH3) , δ 15 N i-NH3(p-NH4+) , or δ 15 N i-NH3(w-NH4+) ; Eq. ( 11 − 13), respectively). δ^15N_i-NH3(a-NH3)=δ^15N_a-NH3-^15 _a-NH3
 (11) 
    δ^15N_i-NH3(p-NH4+)=δ^15N_p-NH4+-^15 _p-NH4+
 (12) 
    δ^15N_i-NH3(w-NH4+)=δ^15N_w-NH4+-^15 _w-NH4+
 (13) We found that differences between δ 15 N i-NH3(a-NH3) and δ 15 N i-NH3(p-NH4+) , δ 15 N i-NH3(a-NH3) and δ 15 N i-NH3(w-NH4+) , δ 15 N i-NH3(p-NH4+) and δ 15 N i-NH3(w-NH4+) are negligible, averaging 0.4 ± 2.3‰, −0.2 ± 1.3‰, and −0.4 ± 2.5‰, respectively (Supplementary Fig. 9 ). This demonstrates that the mean annual 15 ∆ a-NH3 , 15 ∆ p-NH4+ , and 15 ∆ w-NH4+ values (Supplementary Fig. 8 ) estimated by the mean annual f p-NH4+ values (Supplementary Fig. 7 ) can be used to calculate corresponding δ 15 N i-NH3 (Fig. 3b ) of site-based δ 15 N a-NH3 , δ 15 N p-NH4+ , or δ 15 N w-NH4+ (Fig. 3a ) and to estimate the source contributions using the SIAR model. Relative contributions and amounts of v-NH 3 and c-NH 3 emissions Site-based F v-NH3 and F c-NH3 values of each region (Eqs. ( 2 − 4 )) were calculated using the SIAR model [62] . Because each of our calculations has only two end members, the SIAR model can determine the F v-NH3 and F c-NH3 values. Moreover, this model allows us to incorporate isotope effects (by inputting mean annual 15 ∆ a-NH3 , 15 ∆ p-NH4+ , and 15 ∆ w-NH4+ in our calculations; Supplementary Fig. 8 ), the variabilities in δ 15 N of both sources (by inputting mean ± SD of δ 15 N v-NH3 and δ 15 N c-NH3 ; Supplementary Fig. 2b ) and the mixture (by inputting all replicate measurements of δ 15 N a-NH3 , δ 15 N p-NH4+ , or δ 15 N w-NH4+ at each site) into the source contributions. In each run, the percentage data ( n = 10000) output from the SIAR model was used to calculate the mean ± SD values of corresponding F v-NH3 and F c-NH3 at each site, then site-based mean ± SD values of F v-NH3 and F c-NH3 (Supplementary Figs. 10 & 11 ) were used to calculate the mean ± SD values of each region (Fig. 5a ). The mean annual F v-NH3 and F c-NH3 were calculated by inputting all replicate measurements of δ 15 N a-NH3 , δ 15 N p-NH4+ , or δ 15 N w-NH4+ in each year at each site (Fig. 4 ; Supplementary Fig. 12 ). Based on the amount of the v-NH 3 emission ( A v-NH3 ), we calculated corresponding amounts of total NH 3 emissions ( A total , Eq. ( 14 )) and the c-NH 3 emission ( A c-NH3 , Eq. ( 15 )). A_total=A_v-NH3/F_v-NH3
 (14) 
    A_c-NH3=A_total-A_v-NH3
 (15) Regional mean ± SD of A v-NH3 and F v-NH3 were used to calculate regional mean ± SD of A total and A c-NH3 (Fig. 5 ). The annual A c-NH3 (Supplementary Fig. 14a ) was calculated using the mean A v-NH3 (Supplementary Fig. 1a ) and mean ± SD of site-based F v-NH3 values in each year (Supplementary Fig. 12 ). The SDs of A total and A c-NH3 values were propagated errors estimated by using the same MCM described above. Statistical analyses The SPSS 18.0 software package (SPSS Science, Chicago, USA) and Origin 2016 statistical package (OriginLab Corporation, USA) for Windows were used for data analyses in this study. The Tukey honest significant difference (Tukey HSD) and the least significant difference (LSD) tests of the one-way analysis of variance (ANOVA) were used to identify significant differences in δ 15 N among a-NH 3 , w-NH 4 + , and p-NH 4 + (Fig. 3a ), East Asia, North America, and Europe (Fig. 3b ), major sources (Supplementary Fig. 2 ), and urban and non-urban sites or agricultural and non-agricultural sites (Supplementary Fig. 4 ), in F c-NH3 values among East Asia, North America, and Europe (Supplementary Fig. 10 ), and urban and non-urban sites or agricultural and non-agricultural sites (Supplementary Fig. 11a ). Linear regressions were used to examine correlations between sampling years and δ 15 N i-NH3 (Fig. 4 ), 15 ∆ a-NH3 , 15 ∆ p-NH4+ , or 15 ∆ w-NH4+ and f p-NH4+ values (Supplementary Fig. 5 ), f p-NH4+ values and NO x and SO 2 emissions (Supplementary Fig. 6 ), F c-NH3 values at non-urban sites with the corresponding distances from the edge of the nearest urban area (Supplementary Fig. 11b ), sampling years and F c-NH3 or F v-NH3 /F c-NH3 ratio (Supplementary Fig. 12 ), and sampling years and A c-NH3 or A v-NH3 /A c-NH3 ratio (Supplementary Fig. 14 ). Statistically significant differences were set at p < 0.05 or as otherwise stated. The maps with the observation sites for δ 15 N (Fig. 2 ) were plotted with ArcGIS 10.5 software (Esri Inc., USA).